A surface curvature oscillation model for vapour–liquid–solid growth of periodic one-dimensional nanostructures While the vapour–liquid–solid process has been widely used for growing one-dimensional nanostructures, quantitative understanding of the process is still far from adequate. For example, the origins for the growth of periodic one-dimensional nanostructures are not fully understood. Here we observe that morphologies in a wide range of periodic one-dimensional nanostructures can be described by two quantitative relationships: first, inverse of the periodic spacing along the length direction follows an arithmetic sequence; second, the periodic spacing in the growth direction varies linearly with the diameter of the nanostructure. We further find that these geometric relationships can be explained by considering the surface curvature oscillation of the liquid sphere at the tip of the growing nanostructure. The work reveals the requirements of vapour–liquid–solid growth. It can be applied for quantitative understanding of vapour–liquid–solid growth and to design experiments for controlled growth of nanostructures with custom-designed morphologies. Since its first report in 1964 (ref. 1 ), the vapour–liquid–solid (VLS) process has been widely used for synthesizing a wide variety of one-dimensional (1D) materials from micrometre to nanometre in diameter [2] , [3] , [4] , [5] , [6] , [7] , [8] , [9] , [10] , [11] , [12] . 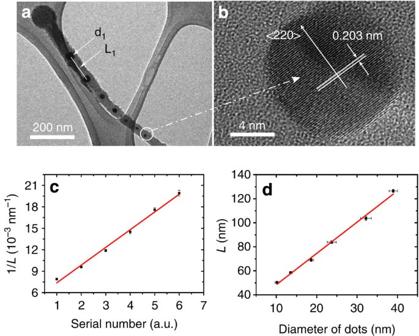Figure 1: Si nanodots obtained by VLS growth without using catalyst. (a) A TEM image of the product. (b) An HRTEM image of a nanodot in (a). (c) Plot of the 1/Lagainst serial number. (d) Plot of diameter of crystal Si nanodots againstL. Error bars represent s.d. In addition to 1D structures with uniform (type a as shown in Table 1 ) and smooth (types a-c) diameters, structures with many other morphologies have been reported. For example, diameter oscillation in VLS-grown Si/SiO 2 core-shell nanowires (type d) has been observed and explained by the Rayleigh instability [6] , [13] . Recently, Oliveira et al . [7] reported periodic diameter oscillations in VLS-grown InP nanowires (type e). They found that the length between each diameter oscillation along the wire depends on the In precursor flow rate during growth. They attributed this periodic growth to a deformation of the triple phase line at the catalyst nanoparticle edge. In contrast, it is interesting that while 1D structures with periodic features (types d–g) are often observed in nanowires, such periodicities are rare in 1D whiskers with diameters of over tens of micrometres. While novel optoelectronic properties due to quantum confinement effects have drawn much attention [14] , [15] , [16] , [17] , [18] , there is less discussion on the possible nanometre size effects on the growth mechanisms of nanostructures [19] . Table 1 1D nanostructures of different morphologies grown with VLS processes. Full size table In this work, we explore the influences of size effects on the periodic growth of 1D nanostructures and noted for the first time that geometries of these periodic nanostructures can be quantitatively described by two linear relations: first, the inverse of the periodic spacing along the wire direction follows an arithmetic sequence; second the periodic spacing in wire direction varies linearly with the diameter of the nanostructures. Although these geometrical relationships have neither been reported nor explained, they are found to be surprisingly general and can satisfactorily describe periodic morphologies in 1D nanostructures reported by various groups [6] , [7] , [8] , [9] , [20] . On the basis of study by Oh et al . [21] and our own observations on the oscillation of the contact angle at the liquid-solid interface, we propose a surface curvature oscillation (SCO) model for the growth of 1D nanostructures with the VLS process. The model provides a quantitative description of the formation of the periodic structures and their associated geometric relationships. It can be applied to quantitatively understand VLS processes and to design experiments for controllable growth of nanostructures with custom-designed morphologies. In particular, understandings based on the present work can be applied to promote or suppress and even control the morphology oscillations in nanowires. General geometrical relationships in VLS nanostructures In our first VLS experiment using a solid SiO source without additional catalyst, we synthesized Si nanodots sequence embedded in an amorphous SiO x shell as shown in Fig. 1a . It is pointed out that, although the Si nanodots come up periodically along the product, as shown later, overall composition of the Si embedded SiOx nanowire roughly keeps the Si:O ratio of 1:1 as in the source. Figure 1b shows a high-resolution transmission electron microscope (HRTEM) image of a Si nanodot, where the interplaner spacing of 0.203 nm corresponds to that of the {220} plane of cubic silicon (CAS number: 7440-21-3). EDX (energy dispersive X-ray) and HRTEM analyses reveal the regions between the nanodots are composed of Si and O with an atomic ratio of roughly 1:1 ( Supplementary Fig. 1 and Supplementary Table 1 ). We also did a separate gravimetric analysis experiment, which suggested that the vapour evaporated from the SiO solid source was basically SiO species with little disproportionation during vapour transportation (details in the Methods section). Figure 1: Si nanodots obtained by VLS growth without using catalyst. ( a ) A TEM image of the product. ( b ) An HRTEM image of a nanodot in ( a ). ( c ) Plot of the 1/ L against serial number. ( d ) Plot of diameter of crystal Si nanodots against L . Error bars represent s.d. Full size image From Fig. 1a , we find two quantitative relationships on analysing geometries of the nanodots. For example, the distance between neighbouring nanodots in Fig. 1a are 127, 104, 84, 69, 59 and 50 nm. Interestingly, the reciprocal of these numbers forms a linearly increasing mathematical sequence that can be fitted well with a starting value of 7.87 × 10 −3 nm −1 and an incremental step of 2.47 × 10 −3 nm −1 (line in Fig. 1c ). Figure 1d further shows that diameter of the nanodot changes linearly with the distance between neighbouring nanodots. Data from more nanowires are shown in the supporting information ( Supplementary Fig. 2 ). We carried out another set of VLS growth of 1D structure by adding indium catalyst. This experiment also gives 1D nanostructure with periodic dots along the wire direction ( Fig. 2a ); their structures differ considerably with those obtained in the first experiment ( Fig. 1a,b ). TEM and EDX studies show that the dots are mostly composed of indium ( Fig. 2b ). No crystalline silicon structure is found in the 1D structures. Interestingly, Fig. 2c,d shows that the two mathematical relationships observed in the previous case can also describe the periodic structure in Fig. 2a , even though the two samples have different microstructures. 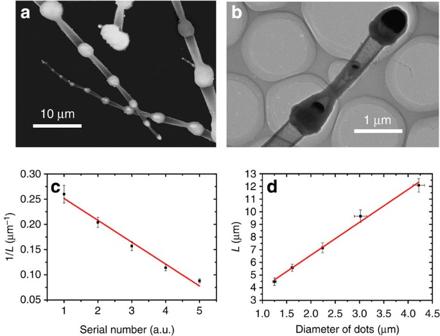Figure 2: SiO nanostructure with In as catalyst in VLS growth. (a) An s.e.m. image of the product. Particles in the background have been de-emphasized in Fig. 2a for clarity (the original image is given inSupplementary Fig. 3). (b) A TEM image of the SiO nanostructures prepared through VLS growth with In catalyst. The tips of the nanowire contain an In metal particle. (c) Plot of 1/Lagainst the serial number. The spherical droplet on the tip of the product is the starting point for the measurement ofLandr.(d) Plot of diameter of dots againstL. Error bars represent s.d. Figure 2: SiO nanostructure with In as catalyst in VLS growth. ( a ) An s.e.m. image of the product. Particles in the background have been de-emphasized in Fig. 2a for clarity (the original image is given in Supplementary Fig. 3 ). ( b ) A TEM image of the SiO nanostructures prepared through VLS growth with In catalyst. The tips of the nanowire contain an In metal particle. ( c ) Plot of 1 /L against the serial number. The spherical droplet on the tip of the product is the starting point for the measurement of L and r. ( d ) Plot of diameter of dots against L . Error bars represent s.d. Full size image We further found that the same mathematical relationships can be used to describe the geometries in 1D nanostructures of other materials systems. For example, periodic geometrical variations in crystalline ZnS nanowires reported by Li et al . [8] can be well described by the two linear relationships ( Supplementary Fig. 4 ). Another example is silica nanofibre bundle reported by Wang et al . ( Supplementary Fig. 5 ) [20] . SCO in VLS processes Diameter oscillation in crystalline InP nanowires has been reported by Oliveira et al . [7] and attributed to changes in the flow rates of reactants. It is interesting that their periodic geometry as shown in the micrograph of type e structure in Table 1 cannot be described by one single equation along the whole length of the nanowires. Nevertheless, the periodic geometries within each local segment can still be described by its own linear relationship ( Supplementary Fig. 6 ). Interestingly, the slope of the linear relation oscillates between negative and positive values of similar magnitudes in alternative segments. The periodic changes in the linear relationship in the alternative segments probably indicate some other oscillations in the macroscopic growth environment such as changes in the flow rates of reactants mentioned by the authors. In the conventional VLS process, the growth kinetic is mainly controlled by the interactions between the vapour phase, the spherical liquid droplet and the solid wire [1] , [2] , [3] . As the spherical tip is the activity centre, we carried out extensive TEM studies on the spherical tips of tens of nanowires from our first experiment. The spherical shape is believed to be inherited from the liquid droplet during VLS growth by the fast quenching experiment in which the growing zone is rapidly quenched from 900 °C to room temperature within 1 s (details in the Methods section). In addition, we found that the spherical tips show three distinct types of morphologies. The tip can contain no ( Fig. 3a ), a half ( Fig. 3b ) or a whole ( Fig. 3c ) silicon particle. Interestingly, the existence of the silicon particle is directly related to the contact angle, θ , between the spherical tip and the stem (defined in Fig. 3a ). The θ in these three cases are in the order of θ a <θ b <θ c as illustrated in Fig. 3 . Judging from the overall wire morphology as shown in Fig. 1a , it is considered that the silicon particles are periodically formed inside the spherical tip and released to the stem along the growth in length. These would imply that the contact angle θ will follow a periodic oscillation consistent with the in situ TEM observation of Kim et al . [19] , [22] and Wen et al . [23] The correlation between Si particles formation with morphology oscillation as well as the precise periodicity shown in Fig. 1a all suggest that Si particles are not formed by random precipitation. Instead, these observations clearly show that formation of Si particles is driven by a morphology-related force. 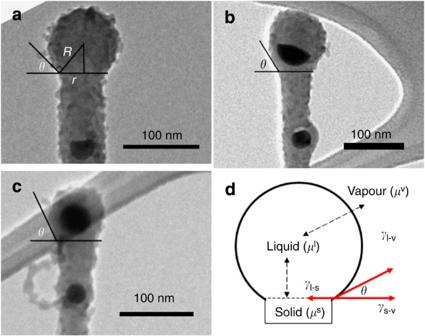Figure 3: The growth tip and VLS processes in it. (a–c) TEM images of the spherical particle at the tip of the nanostructure. Angleθis defined in (a), in whichRandrare, respectively, the radii of the spherical particle and the nanowire. It should be pointed out thatθdefined here is the supplementary angle of the traditionally defined one such as in ref.23. We used the present definition because it leads to much simpler mathematical express in following derivation processes. (d) The growth model of VLS: a nanosize droplet sits on a solid surface surrounded by vapour. Here, the surface tension between the solid and the liquid phase is drawn along the radial direction. It is because oscillation of the wire diameter is controlled by the surface tension and thus movement of the vapour–solid contact point in the radial direction is concerned. Figure 3: The growth tip and VLS processes in it. ( a – c ) TEM images of the spherical particle at the tip of the nanostructure. Angle θ is defined in ( a ), in which R and r are, respectively, the radii of the spherical particle and the nanowire. It should be pointed out that θ defined here is the supplementary angle of the traditionally defined one such as in ref. 23 . We used the present definition because it leads to much simpler mathematical express in following derivation processes. ( d ) The growth model of VLS: a nanosize droplet sits on a solid surface surrounded by vapour. Here, the surface tension between the solid and the liquid phase is drawn along the radial direction. It is because oscillation of the wire diameter is controlled by the surface tension and thus movement of the vapour–solid contact point in the radial direction is concerned. Full size image Considering the geometry as shown in Fig. 3a , the radii of the spherical liquid droplet ( R ) and the wire ( r ) are given by the equation, R=r/ sin θ . As shown in Fig. 1a , r reveals relatively slow change along the wire. The periodic oscillation in θ implies that there should be a corresponding oscillation in R . Pressure inside ( P in ) and outside ( P out ) of the sphere are related by the Young–Laplace equation, where γ l–v is the surface tension at the liquid–vapour interface. Equation (1) suggests that when the liquid droplet is in a nanometre scale, the pressure difference can be significantly modulated by the nanometre size effect ( Supplementary Note 1 ). This implies that for a growth system with a specific external pressure of P out , P in in the liquid sphere would depend strongly on R . When R is small, its oscillation will lead to strong oscillation in P in and thus the kinetic of nucleation and growth of the nanostructures. For the VLS system shown in Fig. 3d at a temperature T and a pressure P out at the deposition zone, if the vapour and liquid phases are in equilibrium, the following condition must be satisfied: . In which, is the chemical potential of the liquid droplet with an equilibrium surface curvature 1 /R e ; and μ v (P out , T) is the chemical potential of the vapour phase at P out and T , respectively. During growth, the actual surface curvature of the droplet 1 /R may be far away from 1 /R e . The droplet will then spontaneously adjusts 1 /R . But it is important to note that the diameter of the growing nanostructure, r , will also vary at the same time. The overall changes on both R and r are linked by R=r/ sin θ , which is governed by the surface tension balance in the system. This is different to the case of a suspended free liquid droplet, which will evaporate if small and continously grow if it is large. For example, we assumed a liquid droplet with a surface curvature 1 /R sits on a nanowire of radius r as shown in Fig. 3d . If 1 /R >1 /R e , the droplet will continuously evaporate because its chemical potential is higher than that of the vapour. But it is important to note that, in the nanowire system, changes in liquid droplet’s volume do not always lead to changes in its diameter in the same direction (that is, a volume decrease might be accompanied with a diameter increase). In fact, this can be well illustrated by the famous coffee ring effect in which evaporation of a coffee droplet leads to decrease in volume but increase in diameter (that is, decrease in curvature) [24] . For example, in the nanowire described in Supplementary Fig. 4 and shown in Fig. 1b of [8] , the nanowire grows with sharp stepwise increase in diameter. This diameter increase might be attributed to the droplet’s diameter increase (that is, liquid–solid boundary expanding) during its volume decrease. In short, the radial growth of nanowire mainly takes place in the period of catalyst droplet evaporation. Eventually, the diameter increase that accompanied with the evaporation would lead to an overshot to R > R e . Now, the droplet’s chemical potential is lower than that of the vapour. Hence, it will adsorb more vapour and lower its chemical potential. This induces a positive feedback in which 1/ R decreases so quickly that the liquid–solid boundary motion is comparatively very slow (growth kinetics shown later in equation (5)). In case that the chosen T , P out and the composition of the vapour are all constant ( Supplementary Note 2 ), and the process is assumed to be isothermal due to the very small droplet size, the actual chemical potential of the liquid is ( Supplementary Discussion ), or where is the actual chemical potential of the liquid droplet for a particular set of θ and r . In these equations, and P ∞ are the chemical potential and the saturated vapour pressure of a liquid phase on a planar surface; V l is the molar volume of the liquid; γ v–l is the surface tension at the vapour–liquid interface; and these are constants for a particular set of growth conditions ( Supplementary Note 3 ). Hence, equation (2) suggests the variation of is a sine function of θ ; while equation (3) reveals it has a linear relationship with 1 /R . However, it should be noted that in the process of 1 /R approaching 1 /R e , part of the liquid would solidify and deposit onto the solid growth surface when its chemical potential is larger than that of the solid phase, because the thermodynamic equilibrium conditions for liquid–solid equilibrium are also dynamically changing with R, r and θ . The liquid volume can decrease by solidification onto the solid nanowire. Indeed, the solidification will be triggered when the chemical potentials between liquid and solid phases satisfy following equation ( Fig. 3d ), where is the liquid phase chemical potential required for solidification; In equation (4), μ s is the chemical potential of the solid phase; A l–s is the areal atom density of the liquid–solid interface;γ s–v is the surface tension at the solid–vapour interfaces; and they are all constants for a particular set of growth conditions ( Supplementary Note 3 ). Equation (4) implies that the required chemical potential for solidification changes following a cosine function of θ . 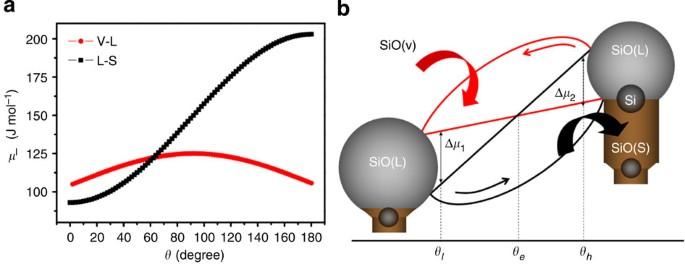Figure 4: The chemical potential oscillation. (a) Numerical simulation plot ofμlagainstθfor a nanowire of 100 nm diameter based on equations (2), (3) and (4) with arbitrarily defined thermodynamic properties. In whichand. (b) VLS growth model of nanowire with a diameter of 100 nm. Figure 4a shows a plot of at different θ for a nanowire of 100 nm in diameter with arbitrarily defined thermodynamic properties ( Supplementary Note 4 ). We now assume that θ at one particular moment during the growth process is 100°. Around the deposition zone of the growth experiment, the chemical potential of the vapour μ v is lower than . Hence, the liquid–solid boundary as well as the r will expand slowly following the Coffee ring effect and which will decrease 1/ R until μ v is higher than . Consequently, the vapour will go into the liquid droplet and trigger a positive feedback process in which 1 /R and thus θ decrease so quickly that the liquid–solid boundary motion is comparatively very slow. In contrast, the liquid will not solidify as . This trend continues until θ approach the intersecting point of , that is, θ e , where the liquid and solid have equal chemical potentials and the solidification becomes energetically feasible. Considering the supersaturation nucleation phenomenon [25] , [26] , we assumed that the liquid in the droplet will only start solidification when ( Fig. 4b ). The solidification would lead to a decrease in R and increases in 1 /R and θ . In contrast, considering undersaturation nucleation [25] , we assume that the solidification will only cease when . Hence, θ will oscillate between θ l and θ h around θ e as shown in Fig. 4b . This directly leads to an oscillation of 1 /R ( Supplementary Note 5 ). Figure 4: The chemical potential oscillation. ( a ) Numerical simulation plot of μ l against θ for a nanowire of 100 nm diameter based on equations (2), (3) and (4) with arbitrarily defined thermodynamic properties. In which and . ( b ) VLS growth model of nanowire with a diameter of 100 nm. Full size image Kinetics of the axis and radial growth in VLS The above thermodynamics analysis reveals that as 1 /R approaches the equilibrium value 1 /R e , it follows an oscillatory instead of a monotonic path. Now we investigate how this SCO modulates nanowire growth by considering growth kinetics. We first consider the evolution of the nanowire’s radius, r . In a nanowire growth experiment, change in r is generally slower than the change in the nanowire’s length, L . In the conventional VLS model, this is explained by considering the relative growth rates of different crystallographic planes [27] , [28] , [29] , [30] . Highly anisotropic growth along the wire direction relative to the radial direction leads to the formation of 1D structures. In contrast, we would like to point out that while the main emphasis of the present work is on the size effects on growth oscillation, there are cases where other factors such as crystallography are important [27] , [28] , [29] , [30] . Theoretically, such crystallography effects could also be considered via the terms μ s and A l–s in equation (4). In other words, equation (4) is valid for both anisotropic and amorphous materials. However, the complexity involved in simultaneous consideration of the size and crystallograph effects is beyond the scope of the present studies and we thus focus on the size effect only. Above all, we would like to point out that the explanation based on crystallographic properties is inadequate for considering growth of amorphous 1D nanowires such as that shown in Fig. 1a . Here, we need a general thermodynamic interpretation on the anisotropic growth. We now consider a situation that vapour is being absorbed into the liquid droplet without spontaneous solidification. The volume increase in the liquid droplet can be accommodated in various ways between two extremes involving changes in R , r and θ . It has to be noted that these three parameters are related by the equation r=R sin θ . In the first extreme, r remains unchanged while R increases and sin θ decreases. In the other extreme, the volume increase is mostly accommodated by a change in r . The main difference between the two extremes is that the liquid–solid interfacial area remains unchanged in the former and increases considerably in the latter case. If the liquid–solid surface tension, γ l–s , is much larger than the liquid–vapour surface tension, γ l–v , the latter case would lead to a much larger surface energy increase. According to the Helmholtz principle of minimum energy dissipation, it can be reasonably expected that the volume increase is accommodated by a way much closer to the former extreme. In other words, when γ l–s >>γ l–v , the nanowire would grow with slow change in r (for example, Fig. 1a ). The nanowire’s axial growth rate d L/ d t is expressed by considering the mass conservation in the liquid droplet: Equation (5) is the Continuity-Equation for fluids, in which V and S are respectively the volume and the surface area of the liquid droplet, while A is surface area of the droplet-wire interface. v v (m s −1 ) is the immigrating speed of vapour atoms into the liquid droplet. It can be seen that axial growth of the wire is suppressed and enhanced, respectively, for d V/ d t > or<0. As discussed above, the nanometre size effect can cause oscillation in R (thus in V ). This implies the wire’s axial growth rate should experience similar oscillation between fast and slow growth. In the extreme case, there can even be oscillation between fast and halted growth that manifested as leapfrog changes in length. In fact, such abrupt solidification/growths have been observed on nanoscale L–S phase transition with in situ microscopies [21] . The above analysis demonstrates that for material systems with thermodynamic properties as described by Fig. 4a , growth of 1D nanostructure would show oscillations in radial direction and leapfrog growth in length direction. The length increase, L , during each oscillation cycle is sum of the length increase during the fast and the slow axial growth. In the Supplementary Discussion , we show that the first term is given by, α · r l ; r l is the radius of the nanowire when the liquid sphere is at the critical supersaturation point where solidification is about to occur. In addition, α depends on θ l and θ h , which are thermodynamic properties of the material system and can be considered as constants under a given temperature and composition. If we define β as the length increase during the slow axial growth step, then, The linear relationship as shown in Figs 1d and 2d , Supplementary Fig. 2 and Supplementary Figs 4–6 can be understood so long as β is much smaller than the first term as suggested by equation (5). The ratios of β/L in the image of Fig. 1b of [8] are 0.15, 0.07, 0.03 and 0.04. The results reveal that except for the cycles with short L , β gives small and diminishing contribution to the growth in length. Energy quantization in VLS growth We now proceed to consider the relationship between L in the n th and the ( n +1)th oscillation cycles. In particular, we consider the same corresponding stage at the two consecutive cycles. For convenience, we choose the critical supersaturation point just before solidification (that is, θ l as shown in Fig. 4b ). According to equation (3), difference in chemical potential of the liquid at the corresponding moment of the two cycles is (Supplementary Discussion), in which and can be considered as constant for the two points. Then we get, equation (8) reveals that can be calculated from the periodic geometry of the nanostructures. As discussed above, for small β , L is approximately proportional to r . We can then write, According to Figs 1c and 2c , equation (9) is valid only if is constant in the corresponding experiment. This requires to be a constant; that is, the change in the chemical potential in each oscillation cycle is about the same. The origin of this might be related to the two-species model for melting-curve maxima that had been found in molten metals such as Ce, Te and intermetallic compounds BbTe 3 et al . [31] , [32] It is now clear that the geometric oscillation and the two linear relationships can be traced back to the liquid droplet’s nanometre size effect on the growth kinetics. In addition to the periodic diameter variation observed in Supplementary Figs 4–6 , it is worth noting that very recently observed catalyst droplet oscillations in straight Ge nanowire growth by using real-time in situ scanning electron microscopy might also be described by the above discussion [33] . However, the situation in our first experiment involves another factor—the coexistence of crystalline silicon nanodots segment and the amorphous SiO segment. We consider this as another evidence of the oscillation cycles. In the silicon suboxide liquid droplet, solidification can occur in two ways. First, amorphous solid can form directly without composition changes. In contrast, disproportionation reaction can occur in which liquid SiO x will be transformed to crystalline Si and amorphous SiO 2 . It is believed that in the present system, the oscillation enables both processes. In particular, the appearance of the crystalline silicon dot is always associated with a smaller R and thus a larger P in . The above analysis reveals the three requirements for the VLS growth: First, the system should be far away from the thermodynamic equilibrium point. Second, the existence of a positive feedback in the growth dynamic as described by equation (3). Finally, the growth oscillation depends on how cross (or not cross) each other as shown in Fig. 4a . Interestingly, these three features of VLS growth match well with those of dissipative structures, provided a new insight into the nanostructure growth. It is worth noting that one application of the present results is to keep the VLS process active for a long time for growing ultra-long single crystal Si nanowire by adjusting the experiment condition to get the leapfrog growth that predicated by equation (5) to take place with high frequency. The ultra-long single-crystal SiNWs have important applications in nanotechnology and thus had been intensively studied, but the longest SiNW reported with evidence is about 2.3 mm according to the best of our knowledge [34] . Bulk preparation of ultra-long single-crystal Si nanowire with an average diameter of 240 nm has been achieved based on VLS growth picture that developed here. As shown in Supplementary Figs 7 and 8 , the ultra-long SiNWs have length of over1.5 cm. In conclusion, the work reveals two quantitative geometric relationships in VLS grown 1D nanostructures. By considering the size effects of the nanoscale catalyst droplet on the chemical potential oscillation of both the V–L and L–S phase transitions, respectively, we demonstrated that a SCO process that drives the VLS growth and quantitatively modulates the morphology of 1D nanostructure with oscillation in the radial direction and leapfrog growth in length direction. It is expected that the simplicity and generality of this model may make it a useful tool for custom engineering of 1D nanostructures with highly controllable geometries. Equipment for nanowire growth The VLS growth was carried out in an alumina (Al 2 O 3 ) tube (Ø=4 cm; L =84 cm) housed in a high-temperature tube furnace ( Fig. 5 ). To freezing the growth in the first experiment, one end of the alumina tube was attached to a quartz tube of 1 cm diameter. A steel rod attached with a magnet on one end is put into the quartz tube such that the rod can be moved with another magnet outside the tube. Temperature distribution along the length of the alumina tube was pre-calibrated using a movable thermometer. 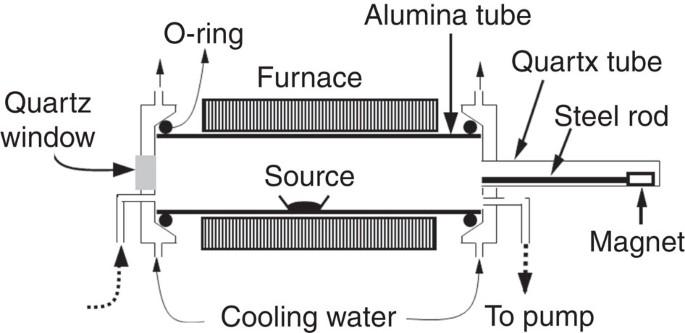Figure 5: Equipment for growing periodic Si nanostructures. Product shown in Figure 1 grows with SiO as source and a moveable steel rod is used. Product shown in Figure 2 grows with SiO and In as source without using the steel rod. Products shown in Figure 6 grow with SiO as source without using the steel rod. Figure 5: Equipment for growing periodic Si nanostructures. Product shown in Figure 1 grows with SiO as source and a moveable steel rod is used. Product shown in Figure 2 grows with SiO and In as source without using the steel rod. 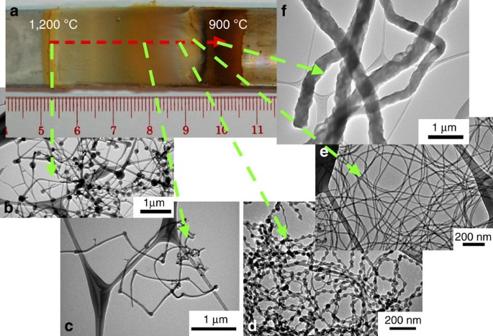Figure 6: Si nanostructures collected at regions of different temperatures. (a) The photo image of the as-prepared sample. (b–f) TEM images of the sample at different temperature regions. The sample is transferred and dispersed in anhydrous alcohol before TEM checking. Products shown in Figure 6 grow with SiO as source without using the steel rod. Full size image Synthesis of nanostructures SiO (Aldrich, 325 mesh, purity>99.9%) powder was loaded in an alumina sample holder. The system was firstly pumped to 5 × 10 −2 mbar and then filled with nitrogen. The SiO powder was heated to 1,350 °C at a pressure of 350 mbar. Many experiments were carried out to maintain the temperature and pressure for different durations. It was observed that growth of nanostructures started abruptly after about 45 min at the region of about 900 °C on various substrates including silicon and alumina. It appears that the growth occurs in a spontaneous manner when the experimental environment reaches a certain critical condition. With this information, we designed an experiment to capture the moment of this spontaneous growth. After holding the experimental conditions for 40 min (that is, shortly before the spontaneous growth), the steel rod was moved into the region of about 900 °C and withdrawn after about 1 s. As the steel rod was maintained at about room temperature before inserting into the hot zone, it functions as a cooling finger to trigger the spontaneous growth of nanostructures. Temperature rise in the steel rod was estimated in a separate experiment, in which the heated rod was immersed into water with known volume and initial temperature. From the temperature rise in the water, masses and specific heat capacities of steel and water, temperature rise in the steel rod was estimated to be about 20±2 °C. An additional growth experiment was carried out at the same temperature and pressure and a growth duration of 90 min. A silicon substrate was put at the region of 900 °C. The main differences are that the source was a mixture of SiO and indium and that the cooling rod was not used. Composition of the evaporated SiO To determine the nature of the species evaporated from the SiO solid source, we did a separate experiment in which Si nanostructures grown with a SiO source without any catalyst were collected from regions of different temperatures ( Fig. 6 ). To obtain enough amounts of samples (about 100 mg) for accurate composition analysis, the growth duration was extended to 6 h. The obtained samples were loaded into alumina crucibles with covers, and accurately weighted before and after further annealing at 1,000 °C in air for complete oxidation. The oxygen contents of the original samples were determined from their weight gains on oxidation. As shown in Table 2 , the Si:O atomic ratios in all samples are approximately 1:1. If the evaporated species from the SiO solid source underwent any disproportionation reaction before deposition, it would be highly unlikely to obtain a uniform composition in the products deposited at different temperature zones. On the basis of this result, we consider that the vapour composition is almost the same along the length in the alumina tube. Figure 6: Si nanostructures collected at regions of different temperatures. ( a ) The photo image of the as-prepared sample. ( b – f ) TEM images of the sample at different temperature regions. The sample is transferred and dispersed in anhydrous alcohol before TEM checking. Full size image Table 2 Gravimetric result of Si nanostructures at different temperatures. Full size table How to cite this article: Wang, H. et al . A surface curvature oscillation model for vapour–liquid–solid growth of periodic one-dimensional nanostructures. Nat. Commun. 6:6412 doi: 10.1038/ncomms7412 (2015).